Small molecules enable neurogenin 2 to efficiently convert human fibroblasts into cholinergic neurons Cell fate can be reprogrammed by modifying intrinsic and extrinsic cues. Here we show that two small molecules (forskolin and dorsomorphin) enable the transcription factor Neurogenin 2 (NGN2) to convert human fetal lung fibroblasts into cholinergic neurons with high purity (>90%) and efficiency (up to 99% of NGN2-expressing cells). The conversion is direct without passing through a proliferative progenitor state. These human induced cholinergic neurons (hiCN) show mature electrophysiological properties and exhibit motor neuron-like features, including morphology, gene expression and the formation of functional neuromuscular junctions. Inclusion of an additional transcription factor, SOX11, also efficiently converts postnatal and adult skin fibroblasts from healthy and diseased human patients to cholinergic neurons. Taken together, this study identifies a simple and highly efficient strategy for reprogramming human fibroblasts to subtype-specific neurons. These findings offer a unique venue for investigating the molecular mechanisms underlying cellular plasticity and human neurodegenerative diseases. Cell fate is determined and maintained by both intrinsic and extrinsic cues [1] . Altering these cues can reprogramme one cell type to another, as demonstrated by the direct conversion of somatic cells into functional neurons through lineage-specific transcription factors [2] , [3] , [4] , [5] , [6] , [7] , [8] , [9] , [10] , [11] , [12] , [13] , [14] , [15] . However, current reprogramming methodologies for human somatic cells require multiple transcription factors and/or microRNAs. This process is generally inefficient and yields specific neuronal subtypes of low purity. Signalling molecules have important roles in cell fate determination and maintenance [1] . We sought to test the hypothesis that these molecules can facilitate transcription factor-mediated reprogramming. We initially focused on Neurogenin 2 (NGN2), a basic helix-loop-helix transcription factor that regulates commitment of neural progenitors to neuronal fate during development and reprogrammes early postnatal astroglia into neurons [14] , [16] , [17] , [18] . NGN2 also has a critical role in specifying motor neuron identity during spinal cord development [19] , [20] , [21] , [22] . However, NGN2 as a key factor has less been employed in neuronal reprogramming from human fetal or adult fibroblasts. Through screening a pool of seven small molecules, we have here defined a culture composition enabling NGN2 to efficiently convert human fetal fibroblasts into pure and functional cholinergic neurons. This basic composition consists of forskolin (FSK), an activator of cAMP signalling, and dorsomorphin (DM, also known as Compound C), an inhibitor of bone morphogenetic protein signalling. SOX11 is an additional factor required for NGN2 to efficiently reprogramme human postnatal and adult fibroblasts to highly pure cholinergic neurons under the defined culture condition. Highly efficient conversion of human fibroblasts into neurons We selected seven small molecules known to target signalling pathways or induce epigenetic changes important for neurogenesis and/or neuronal survival ( Supplementary Table S1 ). Human fetal lung IMR-90 or MRC-5 fibroblasts were transduced with retrovirus expressing NGN2–IRES–GFP and treated individually with these molecules 2 days post retroviral infection (d.p.i.) for 4 days. Transduction efficiency was estimated at 50% by green fluorescent protein (GFP) expression. Over a time course of 22 d.p.i., the neuronal marker Tuj1 was undetected in cultures treated with either vehicle or six of the small molecules. In contrast, FSK treatment resulted in extensive production of Tuj1 + cells with neuronal-like morphology in a dose-dependent manner ( Fig. 1a and Supplementary Fig. S1 ). These cells appeared as early as 7 d.p.i. and survived to 10 d.p.i. However, most of these cells died before developing into MAP2 + mature neurons. Therefore, we screened for additional chemicals to enhance neuronal survival. We found that DM can synergize with FSK to promote both neuronal survival and maturation, although independently DM has no effect on neuronal conversion ( Fig. 1a–c ). Under this defined culture condition, more than 95% of GFP + cells expressed mature neuronal marker MAP2 by 14 d.p.i. In contrast, treatment with other small molecules had either no effect (RA or SB) or inhibited neuronal maturation (VPA, NaB, TSA; Fig. 1c ). Inclusion of a third chemical to the FSK and DM cocktail also failed to further enhance the reprogramming efficiency. 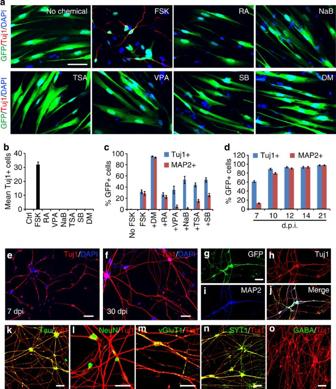Figure 1: NGN2 induces rapid and efficient neuronal conversion of human fetal fibroblasts. (a) FSK but not any other tested small molecules synergizes with NGN2 to generate Tuj1+cells from IMR-90 fetal fibroblasts. GFP indicates cells transduced with NGN2-expressing virus. FSK, forskolin; RA, retinoic acid; VPA, valproic acid; NaB, sodiumn-butyric acid; TSA, trichostatin A; SB, SB431542; DM, dorsomorphin. (b) Quantification of Tuj1+cells 5 days post chemical treatments (means±s.e.m.,n=40 randomly selected × 20 fields from triplicate samples). (c) DM promotes conversion efficiency, neuronal survival and maturation. Cells were counted 10 days post treatment (means±s.e.m.,n=30 random × 20 fields from triplicate samples). (d) Time-dependent maturation of converted neurons by NGN2/FSK/DM (means±s.e.m.,n=10 random × 20 fields from triplicate samples). (e,f) Representative morphology of induced neurons at 7 or 30 d.p.i. (g–l) Converted cells express markers for mature neurons. (m,n) Induced neurons express glutamatergic (vGlut1) and presynaptic (synaptotagmin 1, SYT1) markers, which showed a punctate staining pattern. (o) GABA is rarely detected in converted neurons. Scale bars, 50 μm fora,e–k,n,o, and 20 μm forl,m. DAPI, 4′,6-diamidino-2-phenylindole. Figure 1: NGN2 induces rapid and efficient neuronal conversion of human fetal fibroblasts. ( a ) FSK but not any other tested small molecules synergizes with NGN2 to generate Tuj1 + cells from IMR-90 fetal fibroblasts. GFP indicates cells transduced with NGN2-expressing virus. FSK, forskolin; RA, retinoic acid; VPA, valproic acid; NaB, sodium n -butyric acid; TSA, trichostatin A; SB, SB431542; DM, dorsomorphin. ( b ) Quantification of Tuj1 + cells 5 days post chemical treatments (means±s.e.m., n =40 randomly selected × 20 fields from triplicate samples). ( c ) DM promotes conversion efficiency, neuronal survival and maturation. Cells were counted 10 days post treatment (means±s.e.m., n =30 random × 20 fields from triplicate samples). ( d ) Time-dependent maturation of converted neurons by NGN2/FSK/DM (means±s.e.m., n =10 random × 20 fields from triplicate samples). ( e , f ) Representative morphology of induced neurons at 7 or 30 d.p.i. ( g – l ) Converted cells express markers for mature neurons. ( m , n ) Induced neurons express glutamatergic (vGlut1) and presynaptic (synaptotagmin 1, SYT1) markers, which showed a punctate staining pattern. ( o ) GABA is rarely detected in converted neurons. Scale bars, 50 μm for a , e – k , n , o , and 20 μm for l , m . DAPI, 4′,6-diamidino-2-phenylindole. Full size image We examined the effect of FSK and DM on neuronal induction using 36 additional candidate genes that encode transcription factors and microRNAs ( Supplementary Table S2 ). We did not detect neuron-like Tuj1 + cells under the same culture condition ( Supplementary Fig. S2 ). ASCL1-transduced cells infrequently resulted in Tuj1 + cells. However, these cells showed primitive unipolar or bipolar morphology and did not exhibit mature neuronal features even following extended culture beyond 30 d.p.i. Taken together, these data indicate that FSK and DM uniquely cooperate with NGN2 to reprogramme human fetal fibroblasts to neurons. Functional maturation of human fibroblast-derived neurons A time course analysis of the reprogramming process showed that Tuj1 + cells began to appear at 7 d.p.i. and sharply increased by 10 d.p.i. At 14 d.p.i., a respective 87 and 99% of the surviving NGN2-transduced IMR-90 and MRC-5 cells (indicated by GFP) became Tuj1 + neurons. This represents 56 and 234% of the initially transduced IMR-90 and MRC-5 cells, respectively ( Supplementary Fig. S3a,b ). The induced neurons survived over 30 days with progressive neurite outgrowth ( Fig. 1d–f and Supplementary Fig. S3c ). Transcriptomic analysis at 21 d.p.i. distinctively clusters these induced neurons with neurons of the human brain and spinal cord, but not the parental fibroblasts ( Supplementary Fig. S4a ). Highly enriched gene sets include those involved in neuron projection, synapse formation and synaptic vesicle tethering. In contrast, markers for proliferating fibroblasts, such as genes involved in mitotic spindle formation, extracellular matrix and collagen are dramatically downregulated ( Supplementary Fig. S4b ). The reprogramming process was accompanied by a progressive appearance of neuronal morphology as indicated by round or pyramidal somas, condensed nuclei and growth of multiple neurites and long axons ( Fig. 1f ). Nearly all Tuj1 + cells expressed mature neuronal markers such as MAP2, Tau and NeuN by 14 d.p.i. ( Fig. 1g–l ). After 21 d.p.i., more than 90% of Tuj1 + cells were also positive for glutamatergic (vGLUT1) and presynaptic (SYT1) markers in a stereotypical punctuate pattern ( Fig. 1m ). In contrast, markers for astroglia (GFAP) were undetected ( Supplementary Fig. S5a ) and GABAergic neurons were rarely observed (<0.1%) ( Fig. 1o ; Supplementary Fig. S5b ). Induced neurons cultured for 50 d.p.i. or longer displayed characteristic electrophysiological properties. A train of action potentials was elicited by injecting depolarizing current steps ( Fig. 2a ). Depolarizing voltage steps at −30 mV and above elicited a fast inward, tetrodotoxin (TTX)-sensitive current that resembles current from voltage-dependent sodium channels in primary neurons ( Fig. 2b–e ). A brief puff of GABA, glycine or kainate onto these neurons also activated their respective receptors ( Fig. 2f–h ). Spontaneous synaptic currents were detected when cocultured with cortical neurons ( Fig. 2i ). Subunits of the voltage-gated sodium (Scn3b), potassium (Kcnj6) and calcium (Cacna1h) channels that may serve to generate relevant electrical signals were robustly induced in converted neurons ( Supplementary Fig. S6 ). 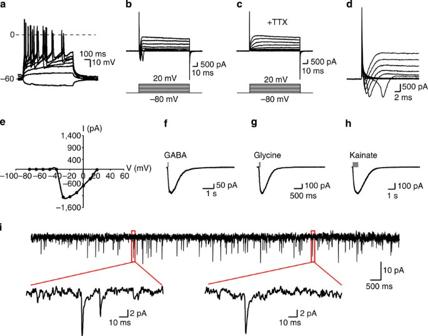Figure 2: NGN2-induced neurons are functionally mature. (a) Fibroblast-derived neurons fire repetitive action potentials by depolarizing current injections (n=10/10 recorded cells). (b,c) TTX-sensitive fast inward currents on depolarization (n=7/7 recorded cells). (d,e) Sodium currents elicited at or above −30 mV, with a peak current at −1,200 pA. (f–h) Inward currents induced by puffing inhibitory or excitatory neurotransmitters (n=3/4 for GABA,n=3/5 for glycine andn=3/3 for kainate). (i) Induced neurons exhibit spontaneous synaptic currents indicating synaptic connections between neurons (n=19/19 of recorded cells). Figure 2: NGN2-induced neurons are functionally mature. ( a ) Fibroblast-derived neurons fire repetitive action potentials by depolarizing current injections ( n =10/10 recorded cells). ( b , c ) TTX-sensitive fast inward currents on depolarization ( n =7/7 recorded cells). ( d , e ) Sodium currents elicited at or above −30 mV, with a peak current at −1,200 pA. ( f – h ) Inward currents induced by puffing inhibitory or excitatory neurotransmitters ( n =3/4 for GABA, n =3/5 for glycine and n =3/3 for kainate). ( i ) Induced neurons exhibit spontaneous synaptic currents indicating synaptic connections between neurons ( n =19/19 of recorded cells). Full size image Direct fate switch of human fibroblasts to neurons While NGN2 expression itself had no major effect on the morphology or cell proliferation of human fetal fibroblasts, the addition of FSK and DM to the culture medium induced rapid morphological changes. This was confirmed by time-lapse live-cell imaging for 120 h post-treatment with small molecules ( Supplementary Fig. S7 ). NGN2-expressing cells (indicated by coexpressed GFP) were elongated 4 h post-treatment and extended neurites by 24 h. These morphological changes were also accompanied by a gradual reduction in cell body size. The majority of NGN2-expressing cells had morphed into neuron-like cells with long bipolar or multipolar processes and a smaller soma-like cell body by 120 h post-treatment. Cell proliferation was rarely observed during live-cell imaging and was further examined by 5-bromodeoxyuridine (BrdU)-labelling experiments ( Fig. 3 ). MRC-5 cells were transduced with retrovirus encoding GFP or NGN2–IRES–GFP and were switched to FSK- and DM-containing induction medium 40 h later. Proliferating cells were pulse-labelled with BrdU (10 μM) for 2 h before immunocytochemical analyses at 24, 48 or 72 h post viral infection (h.p.i. ), respectively ( Fig. 3a ). Around 50% of cells were BrdU-labelled at 24 h.p.i. and this dropped to ~30% one day later. At 72 h.p.i. less than 5% of cells were BrdU-labelled ( Fig. 3b ). Interestingly, no significant difference in the number of BrdU-labelled cells was observed between cells transduced with GFP or NGN2–IRES–GFP, indicating treatment with small molecules rather than NGN2-expression resulted in cell cycle exit. Consistent with cell cycle exit associated with the reprogramming process, converted neurons were rarely labelled even after long-term incubation with BrdU starting from 3 d.p.i. (1 day after treatment with FSK and DM; Fig. 3d–g ). Long-term BrdU-labelling was shown as not toxic, as 70% of the converted neurons could be labelled if BrdU-treatment started 2 days before the addition of FSK and DM. 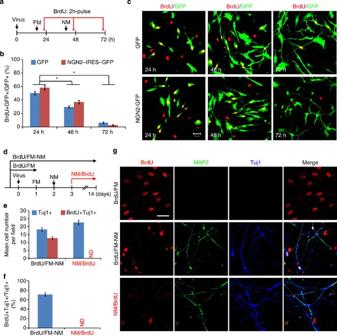Figure 3: Neuronal conversion from human fibroblasts is accompanied by cell cycle exit. (a) Experimental design for data inb,c. Cells were incubated with BrdU for 2 h before immunocytochemistry. FM, fibroblast medium; NM, neuronal induction medium containing FSK and DM. (b,c) Treatment with neuronal induction medium quickly stopped proliferation of cells transduced with either GFP or NGN2–IRES–GFP viruses (means±s.e.m.,n=15 randomly selected × 20 fields from triplicate samples, *P<0.001 by Student’st-test). Scale bar, 50 μm. (d) Experimental design for data ine–g. Cells were treated with BrdU for the indicated periods of time. (e–g) A majority of the cells were labelled with BrdU if treated before neuronal conversion (BrdU/FM-NM), whereas cells were not labelled by BrdU if treated 1 day after switching to neuronal induction medium (NM/BrdU). Quantitative data are means±s.e.m. from 20 randomly selected × 20 fields from triplicate samples. ND, not detected. Scale bar, 50 μm. Figure 3: Neuronal conversion from human fibroblasts is accompanied by cell cycle exit. ( a ) Experimental design for data in b , c . Cells were incubated with BrdU for 2 h before immunocytochemistry. FM, fibroblast medium; NM, neuronal induction medium containing FSK and DM. ( b , c ) Treatment with neuronal induction medium quickly stopped proliferation of cells transduced with either GFP or NGN2–IRES–GFP viruses (means±s.e.m., n =15 randomly selected × 20 fields from triplicate samples, * P <0.001 by Student’s t -test). Scale bar, 50 μm. ( d ) Experimental design for data in e – g . Cells were treated with BrdU for the indicated periods of time. ( e – g ) A majority of the cells were labelled with BrdU if treated before neuronal conversion (BrdU/FM-NM), whereas cells were not labelled by BrdU if treated 1 day after switching to neuronal induction medium (NM/BrdU). Quantitative data are means±s.e.m. from 20 randomly selected × 20 fields from triplicate samples. ND, not detected. Scale bar, 50 μm. Full size image Time course analysis of gene expression by quantitative reverse transcription–polymerase chain reaction (qRT–PCR) showed that Sox2 , Olig2 and Pax6 were not detectable during the entire reprogramming process ( Supplementary Fig. S8a–c ). Immunocytochemistry using antibodies specific to SOX1, SOX2 and OLIG2 also showed a lack of specific staining for these markers of neural progenitors ( Supplementary Fig. S8d,e ). Together, these data indicate that neuronal conversion of human fibroblasts by NGN2 and small molecules is direct without passing through a proliferative progenitor intermediate. Neuronal conversion without long-term expression of NGN2 qRT–PCR analysis revealed an induction of endogenous NGN2 and a dramatic downregulation of retroviral NGN2 beginning at 14 d.p.i. ( Fig. 4a ). We used a doxycycline (Dox)-inducible system to control NGN2 expression and examined total surviving neurons at 35 d.p.i. to temporally characterize the requirement for exogenous NGN2 ( Fig. 4b–d ). Quantitative analysis of gene expression showed that Dox-induced NGN2 returned to the basal level by 7 days on Dox withdrawal ( Fig. 4c ). Interestingly, human fetal fibroblasts can be reprogrammed into neurons after only 2 days of induced NGN2 expression. The number of neurons increased with longer induction periods and reached a plateau at 21 days ( Fig. 4d ). In total, these data indicate that long-term expression of exogenous NGN2 is not required for neuronal conversion and survival following reprogramming. 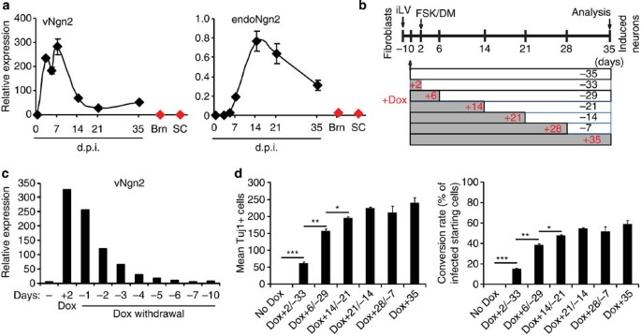Figure 4: Neuronal conversion from human fibroblasts does not require long-term expression of NGN2. (a) qRT–PCR analysis of retrovirus-expressed NGN2 (vNGN2) and the induction of endogenous NGN2 (endoNGN2) at the indicated time points after retroviral transduction of human fetal fibroblasts (means±s.e.m.,n=3 at each time point). Samples from normal adult human brain (Brn) and spinal cord (SC) were used as controls (n=1). (b) Experimental design using doxycycline (Dox) inducible expression system. Cells (5,000/well in 48-well plate) were co-transduced with lentivirus constitutively expressing rtTA3G and Dox-inducible lentivirus expressing NGN2–IRES–GFP under the TRE3G promoter. One day post transduction, Dox (0.1 μg ml−1) was applied for the indicated periods of time and then withdrawn. The transduction efficiency was about 8% indicated by initial GFP expression. Tuj1-expression was analysed 35 days later. (c) qRT–PCR analysis of exogenous NGN2 expression, which returns to basal level 6 days after Dox withdrawal (n=1). (d) NGN2 expression is no longer required after neuronal conversion at 21 d.p.i., although it increases total number of converted neurons at earlier time points. Tuj1+cells were quantified from a whole well from triplicate samples (means±s.e.m.,n=3). *P=0.04, **P=0.003, and ***P=0.0003 by Student’st-test. Figure 4: Neuronal conversion from human fibroblasts does not require long-term expression of NGN2. ( a ) qRT–PCR analysis of retrovirus-expressed NGN2 (vNGN2) and the induction of endogenous NGN2 (endoNGN2) at the indicated time points after retroviral transduction of human fetal fibroblasts (means±s.e.m., n =3 at each time point). Samples from normal adult human brain (Brn) and spinal cord (SC) were used as controls ( n =1). ( b ) Experimental design using doxycycline (Dox) inducible expression system. Cells (5,000/well in 48-well plate) were co-transduced with lentivirus constitutively expressing rtTA3G and Dox-inducible lentivirus expressing NGN2–IRES–GFP under the TRE3G promoter. One day post transduction, Dox (0.1 μg ml −1 ) was applied for the indicated periods of time and then withdrawn. The transduction efficiency was about 8% indicated by initial GFP expression. Tuj1-expression was analysed 35 days later. ( c ) qRT–PCR analysis of exogenous NGN2 expression, which returns to basal level 6 days after Dox withdrawal ( n =1). ( d ) NGN2 expression is no longer required after neuronal conversion at 21 d.p.i., although it increases total number of converted neurons at earlier time points. Tuj1 + cells were quantified from a whole well from triplicate samples (means±s.e.m., n =3). * P =0.04, ** P =0.003, and *** P =0.0003 by Student’s t -test. Full size image Converted cells are highly pure cholinergic neurons Interestingly, the converted neurons have a distinctive morphology resembling that of motor neurons ( Fig. 1f ). At 21 d.p.i., immunocytochemistry and qRT–PCR analysis for converted neurons showed specific expression of motor neuron markers including HB9 (91.7% of neurons, n =325) and ISL1/2 (90.2%, n =347), which specify motor neuron identity. ChAT (choline acetyltransferase, 98.5%, n =325) and VAChT (vesicular acetylcholine transporter, 98.2%, n =273), markers for the production and transport of acetylcholine (ACh, neurotransmitter employed by cholinergic motor neurons), were also robustly expressed ( Fig. 5a–d ). We therefore designated these converted neurons as hiCNs). 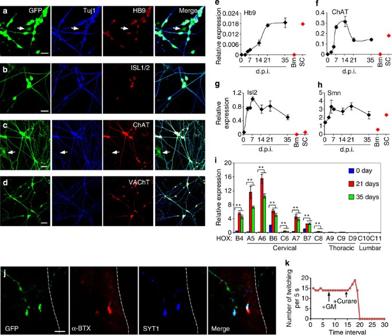Figure 5: Cholinergic motor neuron-like cells converted from human fetal fibroblasts. (a-d) Immunocytochemistry analysis of induced neurons with markers for cholinergic motor neurons, including HB9 (91.7%,n=325), ISL1/2 (90.2%,n=347), ChAT (98.5%,n=325) and VAChT (98.2%,n=273). GFP expression indicates NGN2-transduced cells. Control virus-transduced fibroblasts were stained negative for each of these markers. Arrows indicate cells stained negative for HB9 or ChAT. (e–i) Gene expression analysis by qRT–PCR during the reprogramming process (means±s.e.m.,n=3 at each time point). It was normalized to that of housekeeping geneHprt. Samples from normal adult human brain (Brn) and spinal cord (SC) were used as controls (n=1). **P<0.01 by Student’st-test. (j) Immunocytochemistry analysis of synaptic connections between hiCNs and myotubes in coculture. A multinucleated myotube is outlined. α-BTX, α-bungarotoxin; SYT1, synaptotagmin 1. (k) Quantification of rhythmic contractions of myotubes after coculturing with hiCNs. Such contractions can be blocked by curare, a competitive inhibitor of acetylcholine receptor (n=5 independent myotubes). Scale bars: 20 μm fora,b; 50 μm forc,d; and 10 μm forj. Figure 5: Cholinergic motor neuron-like cells converted from human fetal fibroblasts. ( a - d ) Immunocytochemistry analysis of induced neurons with markers for cholinergic motor neurons, including HB9 (91.7%, n =325), ISL1/2 (90.2%, n =347), ChAT (98.5%, n =325) and VAChT (98.2%, n =273). GFP expression indicates NGN2-transduced cells. Control virus-transduced fibroblasts were stained negative for each of these markers. Arrows indicate cells stained negative for HB9 or ChAT. ( e – i ) Gene expression analysis by qRT–PCR during the reprogramming process (means±s.e.m., n =3 at each time point). It was normalized to that of housekeeping gene Hprt . Samples from normal adult human brain (Brn) and spinal cord (SC) were used as controls ( n =1). ** P <0.01 by Student’s t -test. ( j ) Immunocytochemistry analysis of synaptic connections between hiCNs and myotubes in coculture. A multinucleated myotube is outlined. α-BTX, α-bungarotoxin; SYT1, synaptotagmin 1. ( k ) Quantification of rhythmic contractions of myotubes after coculturing with hiCNs. Such contractions can be blocked by curare, a competitive inhibitor of acetylcholine receptor ( n =5 independent myotubes). Scale bars: 20 μm for a , b ; 50 μm for c , d ; and 10 μm for j . Full size image Notably, the expression of genes for cholinergic motor neurons could be detected as early as 5 d.p.i. reaching a peak between 14 and 21 d.p.i. ( Fig. 5e–g ). SMN , a gene critical for the survival of motor neurons, was also upregulated ( Fig. 5h ). Markers for upper motor neurons [23] , [24] (Fezf2) were not detected ( Supplementary Fig. S9 ). In contrast, Hox gene expression profiles indicated that the induced motor neuron-like cells have a cervical identity [25] , [26] , [27] , [28] , [29] ( Fig. 5i ). After replating, the survival of these neurons also depended on a set of neurotrophic factors (BDNF, GDNF and NT3) essential to motor neurons [30] ( Supplementary Fig. S10 ). These hiCNs maintained their motor neuron-like identity and displayed typical electrophysiological properties 4 weeks after turning off exogenous NGN2 expression ( Supplementary Fig. S11 ). We cocultured hiCNs with C2C12-derived myotubes to assess synaptic functionality. During coculture, hiCN axons extended to form synaptic-like structures innervating the myotubes ( Supplementary Fig. S12a–d ). Staining with α-bungarotoxin revealed clustered ACh receptors on myotubes in close contact with enlarged SYT1 + axonal terminals of hiCNs. This is indicative of the formation of neuromuscular junctions ( Fig. 5j ). Interestingly, myotubes frequently started to contract rhythmically 4–7 days post coculture with hiCNs ( Supplementary Movie 1 ). Incubation with curare, a competitive antagonist of nicotinic ACh receptors, completely blocked hiCN-induced myotube contractions ( Fig. 5k and Supplementary Fig. S12e ). Although myotubes cultured alone or with hiCN-conditioned medium occasionally showed spontaneous contractions, they were discontinuous, arrhythmic and insensitive to curare treatment. Collectively, these data indicate that hiCNs exhibit motor neuron-like functionality. Conversion of adult human fibroblasts into cholinergic neurons We next applied these reprogramming conditions to postnatal and adult skin fibroblasts from 3 to 37-year-old donors ( Supplementary Table S3 ). However, neurons were generated at low efficiency suggesting requirement of an additional factor(s) ( Fig. 6a ). When NGN2 was combined with each of 36 additional candidate genes, only SOX11 greatly potentiated neuronal conversion from fetal ( Supplementary Fig. S13 ), postnatal and adult fibroblasts ( Fig. 6a ). We also screened for additional chemicals or growth factors and found that FGF2 could dramatically enhance reprogramming efficiency ( Fig. 6a ). These data are consistent with a well-established role of SOX11 and FGF2 in neurogenesis, neuronal survival and maturation [31] , [32] , [33] , [34] , [35] , [36] , [37] . Notably, the omission of any of these identified molecules dramatically reduced reprogramming efficiency ( Supplementary Fig. S14 ). 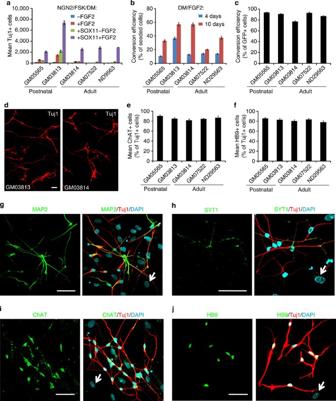Figure 6: Efficient generation of cholinergic neurons from postnatal and adult human skin fibroblasts. (a) SOX11 and FGF2 facilitate NGN2 to convert postnatal (GM05565 and GM03813) or adult (GM03814, GM07522 and ND29563) human skin fibroblasts into neurons. Tuj1+cells were quantified from triplicate samples at 21 d.p.i. (means±s.e.m.). (b,c) Conversion efficiency normalized to total number of seeded cells (b) or NGN2-expressing cells (c). The total number of Tuj1+cells from triplicate samples was quantified at 21 d.p.i. (means±s.e.m.). A longer treatment of DM/FGF2 enhances conversion efficiency. (d) Representative images of converted Tuj1+neurons from postnatal (GM03813) and adult (GM03814, the mother of GM03813) fibroblasts at 21 d.p.i. (e,f) Quantification of converted neurons expressing ChAT (e, 81.9–90.7%) or HB9 (f, 78.0–85.9%). The total number of Tuj1+, ChAT+or HB9+cells from triplicate samples was quantified at 21 d.p.i. (means±s.e.m.). (g–j) Induced neurons from skin fibroblasts (GM07522) express pan-neuronal marker MAP2 (g) and presynaptic marker SYT1 (h). (i,j) Converted neurons from skin fibroblasts (GM03813) are cholinergic (ChAT+,i) and express markers for early motor neurons (HB9+,j). Arrows show cells stained negative for the indicated neuronal markers. Scale bars, 50 μm. DAPI, 4′,6-diamidino-2-phenylindole. Figure 6: Efficient generation of cholinergic neurons from postnatal and adult human skin fibroblasts. ( a ) SOX11 and FGF2 facilitate NGN2 to convert postnatal (GM05565 and GM03813) or adult (GM03814, GM07522 and ND29563) human skin fibroblasts into neurons. Tuj1 + cells were quantified from triplicate samples at 21 d.p.i. (means±s.e.m.). ( b , c ) Conversion efficiency normalized to total number of seeded cells ( b ) or NGN2-expressing cells ( c ). The total number of Tuj1 + cells from triplicate samples was quantified at 21 d.p.i. (means±s.e.m.). A longer treatment of DM/FGF2 enhances conversion efficiency. ( d ) Representative images of converted Tuj1 + neurons from postnatal (GM03813) and adult (GM03814, the mother of GM03813) fibroblasts at 21 d.p.i. ( e , f ) Quantification of converted neurons expressing ChAT ( e , 81.9–90.7%) or HB9 ( f , 78.0–85.9%). The total number of Tuj1 + , ChAT + or HB9 + cells from triplicate samples was quantified at 21 d.p.i. (means±s.e.m.). ( g – j ) Induced neurons from skin fibroblasts (GM07522) express pan-neuronal marker MAP2 ( g ) and presynaptic marker SYT1 ( h ). ( i , j ) Converted neurons from skin fibroblasts (GM03813) are cholinergic (ChAT + , i ) and express markers for early motor neurons (HB9 + , j ). Arrows show cells stained negative for the indicated neuronal markers. Scale bars, 50 μm. DAPI, 4′,6-diamidino-2-phenylindole. Full size image We also found that extending the DM/FGF2 treatment from 4 days to 10 days greatly increased the conversion rate of all fibroblasts examined ( Fig. 6b ), though the continuous presence of these molecules were not necessary after 10 days. Under this condition, 20.3–57.2% of seeded fibroblasts were converted into Tuj1 + neurons at 21 d.p.i. ( Fig. 6b ). When normalized to the number of transduced NGN2-expressing cells, the conversion rate was 77–93% ( Fig. 6c ). The variable rate of viral transduction and heterogeneous nature of donor-derived primary fibroblasts are plausible contributors to this range of conversion efficiencies. Remarkably, induced neurons could be robustly generated from skin biopsies of patients with spinal muscular atrophy (GM03813, 90.8% of NGN2-expressing cells and 57.2% of seeded cells) or amyotrophic lateral sclerosis (ND29563, 87% of NGN2-expressing cells and 37.5% of seeded cells; Fig. 6b–d ), suggesting that these disease conditions did not impede neuronal conversion. The converted neurons expressed Tuj1, MAP2 and SYT1 ( Fig. 6g ). Consistent with a cholinergic phenotype of fetal hiCNs, the majority of postnatal and adult skin fibroblast-derived neurons also expressed ChAT (81.9–90.7%) and HB9 (78.0–85.9%), indicating that the addition of SOX11 and FGF2 did not alter the subtype of the converted neurons ( Fig. 6e ). The ability of directly converting non-neuronal somatic cells into neurons provides a unique opportunity to understand cellular plasticity and model human neurodegenerative diseases in culture. A critical prerequisite to achieving these goals is the high-efficiency generation of a relatively homogenous population of subtype-specific neurons. Yet, the majority of currently available methods have not achieved this standard, especially in models of adult or diseased human cells. For example, motor neuron-like cells were previously generated from human embryonic stem cell-derived fibroblasts; however, as many as eight transcription factors were required and the efficiency was extremely low [4] (<0.05% of the seeded cells). Screening combinations of intrinsic and extrinsic factors with potential synergistic roles in cell fate specification, we unexpectedly found that a combination of two small molecules enables the single transcription factor NGN2 to efficiently convert human fetal fibroblasts into highly pure cholinergic neurons. Inclusion of an additional transcription factor, SOX11, also efficiently converts postnatal and adult human fibroblasts into similarly pure cholinergic neurons. A different combination of small molecules was previously used for cellular reprogramming of stably transduced human fibroblasts by ASCL1 and NGN2 (ref. 2 ). The conversion efficiency is high, but the resulting culture was a mixture of GABAergic (20%), glutamatergic (35%) and a low percentage of other subtype-specific neurons. Intriguingly, none express ChAT or HB9 (ref. 2 ). In stark contrast, our converted neurons from fetal, postnatal and adult human fibroblasts exhibit motor neuron-like cholinergic features with a majority expressing ChAT (81.9–98.5%) and HB9 (78.0–91.7%). Several differences between our protocol and that by Ladewig et al. [2] might explain the specific induction of different neuronal subtypes. First, Ladewig et al. [2] used two factors, ASCL1 and NGN2, which have opposing roles in cell fate determination in different brain and spinal cord regions [38] , [39] . The final balance of these two opposing factors within a heterogeneous cell population might underlie the induction of a mixture of neuronal subtypes. In contrast, our use of a single-cell fate-specifying factor (NGN2) in fetal fibroblasts would activate a cohesive pathway that determines a more homogenous neuronal subtype. As SOX11 only promotes neuronal survival and maturation but does not specify neuronal subtype [31] , [35] , [40] , its inclusion in our protocol for reprogramming postnatal and adult fibroblasts does not change the neuronal subtype that is specified by NGN2. Second, in addition to bone morphogenetic protein/SMAD signalling inhibitors (noggin and LDN-193189), Ladewig et al. [2] also included SB431542, an Activin/Nodal/TGFβ pathway inhibitor, and CHIR99021, a GSK3β inhibitor, in their culture medium [2] . It has been previously shown that GSK3β is critical for phosphorylation of NGN2 and that this phosphorylation regulates motor neuron specification [21] . Indeed, when CHIR99021 was included in our defined condition, HB9 was no longer detectable. These data clearly show the pivotal effect of different combinations of small molecules with different transcription factors on neuronal conversion, confirming decades of research on neural development showing that neuronal identity is specified and tightly maintained by a unique combination of intrinsic and extrinsic cues. Nonetheless, additional factors might be required to further enhance the motor neuron-like phenotype of our hiCNs, as Isl1 and Lhx3 , two transcription factors important for motor neuron specification [41] were undetected by qRT–PCR analysis. In summary, our results show that highly pure subtype-specific neurons can be directly converted from human fibroblasts by the coordinated action of transcription factor(s) and extrinsic cues. This is also the first case demonstrating that NGN2 as a key transcription factor, in combination with the synergistic action of two small molecules, is capable of very efficiently reprogramming human fibroblasts to cholinergic neurons under a defined culture condition. Our high-efficiency reprogramming methodology provides a novel model to tease out the detailed molecular mechanisms underlying cell fate plasticity. Further optimization of the reprogramming process to obtain a homogenous population of cholinergic motor neurons from patients’ fibroblasts will significantly expedite the molecular genetic analysis of motor neuron diseases such as spinal muscular atrophy and amyotrophic lateral sclerosis. These induced patient-specific cholinergic neurons may also provide the most relevant cell type for drug screening and testing. One limitation of direct lineage reprogramming is the scalability of these cells for broader applications. This limitation might be overcome by the expansion of fibroblasts or the derivation of renewable neural stem cells [42] , [43] , [44] , [45] , [46] . The strategy defined here also offers a straightforward method for the discovery of novel combinations of small molecules and transcription factors for improved efficiency in reprogramming somatic cells to proliferative stem cells or other postmitotic cell lineages. Plasmid construction and virus production Complementary DNA of each candidate factor ( Supplementary Table S2 ) was individually subcloned into a retroviral vector (pLNCX2, Clontech). To monitor NGN2-expressing cells, an IRES–GFP or IRES–GFP–T2A–Sox11 cassette was inserted right after the stop codon of the NGN2 gene in plasmid pLNCX2. For Dox-inducible expression, NGN2–IRES–GFP was subcloned into a Dox-inducible lentiviral vector under the control of pTRE3G [pLenti CMVTRE3G eGFP Puro (w819-1), Addgene] promoter. pLenti CMV rtTA3G Blast (R980-M38-658) was obtained from Addgene. Replication-incompetent retroviruses were produced in GP293 cells (Clontech) via calcium phosphate-mediated transfection of CMV–VSV-G and retroviral vectors. Similarly, lentiviruses were generated in HEK293 cells (ATCC) after co-transfection of lentiviral vector, pREV, pMDL and pVSV-G. Cell culture Human fibroblasts were obtained from commercial sources ( Supplementary Table S3 ) and maintained in fibroblast medium (DMEM supplemented with 10 or 15% fetal bovine serum and penicillin/streptomycin) according to the vendor’s instructions for cell culture. Cells were seeded onto gelatin-, fibronectin- or Matrigel-coated culture vessels (4.8 × 10 5 per 24- or 48-well plate or 8 × 10 5 per 10-cm dish) with or without glass coverslips. They were transduced the next day with retroviral supernatants in the presence of 6 μg ml −1 polybrene. After overnight incubation, culture media were refreshed. One day later, the cells were then switched to C2 medium, which consists of DMEM:F12:Neurobasal (2:2:1), 0.8% N-2 (Invitrogen), 0.4% B-27 (Invitrogen), and penicillin/streptomycin. Screens for small molecules were conducted by incubating the indicated chemicals ( Supplementary Table S1 ) in C2 medium for 5 days starting at 2 d.p.i. The resulting neural induction medium for human fetal fibroblasts consist of DM (1 μM, from 2 to 6 d.p.i.) and FSK (10 μM) in C2 medium. For postnatal and adult human fibroblasts, FGF2 (10 ng ml −1 ) and DM was included in the above induction medium from 2 to 12 d.p.i. Induction medium was half-changed every other day. For inducible expression, cells were transduced overnight with lentiviruses. The day after medium change, Dox (0.1 μg ml −1 ) was added to induce gene expression for the indicated period of time during the course of reprogramming. For gene expression analysis, electrophysiology, or coculture with myotubes, induced neurons were purified by differential plating. Briefly, cells at 14–21 d.p.i. were rinsed with Dulbecco's phosphate-buffered saline and dissociated with 0.025% trypsin for 15 min at 37 °C. After blocking trypsin activity with FBS-containing fibroblast medium, the cell suspension was plated onto a gelatin-coated culture dish, to which fibroblasts tightly attached. About 30 min later, floating cells, which mainly consisted of induced neurons, were replated onto a new coated dish to remove residual fibroblasts or were directly collected by centrifugation at 500 g for 2 min. Cells were resuspended into C2 medium and centrifuged again to remove cell debris. Finally, cells were plated onto a coated dish in C2 medium supplemented with BDNF, GDNF and NT3 (10 ng ml −1 each, Peprotech). Unless indicated otherwise, C2 media with neurotrophic factors were half-changed twice a week. The human neural stem cell line, K048, was a kind gift of Dr P. Wu (UT Medical Branch) and Dr C.N. Svendsen (University of Wisconsin). Immunofluorescence, BrdU labelling and cell counting After fixation with 4% paraformaldehyde in PBS for 15 min at room temperature, cells were permeabilized and blocked with blocking solution (1 × PBS containing 0.2% Triton X-100 and 3% BSA) for 1 h. Primary antibodies in blocking solution were then added and incubated overnight at 4 °C, followed by washing and incubation with fluorophore-conjugated corresponding secondary antibodies. Proliferating cells were labelled by BrdU (10 μM) for 2 h or throughout the culture, as indicated. BrdU-incorporation was detected as previously described [47] . Briefly, paraformaldehyde-fixed cells were treated with 2 M HCl for 30 min at 37 °C, rinsed in 0.1 M boric acid for 10 min, and blocked with blocking solution. This was followed by incubation with primary and secondary antibodies. The following antibodies were used: rabbit anti-NGN2 (Chemicon, 1:500), rabbit or mouse anti-Tuj1 (Covance, 1:20,000), mouse anti-MAP2 (Sigma, 1:750), chicken anti-Tau (AVES, 1:500), mouse anti-NeuN (Chemicon, 1:500), mouse anti-vGluT1 (UC Davis, 1:100), mouse anti-synaptotagmin 1 (SYT1, DSHB, 1:200), rabbit anti-GABA (Sigma, 1:2,000), rabbit anti-SOX1 (Cell Signaling, 1:100), rabbit anti-SOX2 (Chemicon, 1:500), rabbit anti-OLIG2 (Millipore, 1:500), mouse anti-BrdU (Sigma, 1:2,000), mouse anti-HB9 (DSHB, 1:100), mouse anti-ISL1/2 (DSHB, 1:100), mouse anti-VAChT (DSHB, 1:200), goat anti-ChAT (Chemicon, 1:200), and Alexa Fluor-conjugated secondary antibodies made in donkey (Invitrogen, 1:500). Images were obtained with a Carl Zeiss LSM510 Confocal Microscope or an Olympus BX51 Microscope equipped with StereoInvestigator software (MBF Bioscience). After counting the total number of Tuj1 + cells within the entire well of a 24- or 48-well plate in triplicate, conversion efficiency was calculated by normalizing to the number of plated cells or to the number of surviving GFP + cells. Transcriptome and qRT–PCR analysis Total RNAs from the indicated samples were isolated by using TRIzol Reagent (Invitrogen) and an RNA extraction kit (Zymo Research). Total RNAs from a 43-year-old healthy human and whole human brain and pooled total RNAs from 20- to 59-year-old healthy human were purchased from Clontech. Gene expression profiling using Human HT-12 v4 BeadChip (Illumina) was performed by the Microarray Core Facility at UT Southwestern. Data with an average fold change of 2 at P ≤0.05 for each comparison were considered for gene ontology analysis by DAVID ( http://david.abcc.ncifcrf.gov/ ). qRT–PCR using independent RNA samples in triplicate was performed using SYBR Green chemistry (Invitrogen). Primer sequences are listed in Supplementary Table S4 . Electrophysiology Reprogrammed neurons, cultured on astrocyte- or cortical neuron-coated glass coverslips for 4–6 weeks, were used for analysis. Whole-cell recordings were made under visual guidance using infra-red differential interference contrast (IR-DIC) and GFP-fluorescence to identify GFP + cells. For recordings with inducible expression of NGN2, converted neurons at 21 d.p.i. were labelled with DiI (2 μg ml −1 , Invitrogen), washed, and plated on astrocyte-coated coverslips in Dox-free neuronal culture medium. Recordings on DiI + GFP - cells were conducted 29 days later. Recordings were made at 30 °C in a submersion chamber perfused at 3 ml min −1 with artificial cerebrospinal fluid containing: 119 mM NaCl, 2.5 mM KCl, 26 mM NaHCO 3 , 1 mM NaH 2 PO 4 , 11 mM D -glucose, 3 mM CaCl 2 , and 2 mM MgCl 2 at pH 7.28, 300 mOsm and saturated with 95%O 2 /5%CO 2 . Whole-cell recordings were performed on induced neurons using recording pipettes (approximately 3–5 MΩ) filled with an intracellular solution containing: 0.2 mM EGTA, 130 mM K-Gluconate, 6 mM KCl, 3 mM NaCl, 10 mM HEPES, 4 mM ATP-Mg, 0.4 mM GTP-Na, 14 mM phosphocreatine-di(Tris) at pH 7.2 (adjusted by KOH) and 285 mOsm. For GABA and glycine puffing experiments, patch recording pipettes were filled with an intracellular solution containing: 135 mM KCl, 5 mM EGTA, 0.5 mM CaCl 2 , 1 mM MgCl 2 , 10 mM HEPES, 4 mM ATP-Mg, 0.4 mM GTP-Na, 14 mM phosphocreatine-di(Tris) at pH 7.2 and 285 mOsm. Series and input resistance were measured in voltage clamp with a 400 ms, 10 mV step from a −60 mV holding potential (filtered at 30 kHz, sampled at 50 kHz). Cells were only used for analysis if the series resistance was less than 30 MΩ and was stable throughout the experiment. Input resistance ranged from 0.6 to 2 GΩ. Currents were filtered at 3 kHz, acquired and digitized at 10 kHz on a PC using custom software (Labview; National Instruments). Action potentials were recorded in current clamp and elicited by a series of current injections ranging from −20 to 200 pA at 20 pA increments and 400 ms in duration. Sodium currents were recorded in voltage clamp in response to a series of voltage steps ranging from −80 to 20 mV at 10 mV increments and 100 ms in duration according to standard protocols. TTX (1 μM), a voltage-dependent Na + channel blocker, was then applied to the chamber for 8 min and the voltage step was repeated to observe the TTX-sensitive currents. GABA, glycine or kainate (1 μM each) were dissolved in artificial cerebrospinal fluid and puffed onto neurons using a picospritzer III (Parker Instrumentation) with 6–9 psi and 100 ms duration for GABA and glycine or 800 ms duration for kainate. The puffing pipette tip was ~3 MΩ and placed ~10 μm away from the recorded neuron. Induced neurons (identified by GFP or DiI) were cocultured with mouse cortical neurons for the recording of spontaneous synaptic currents. Spontaneous synaptic currents were recorded in voltage clamp. Currents elicited by neurotransmitter puffs were measured in voltage clamp for 6–10 s. In all voltage clamp recordings, cells were clamped at −60 mV except during the voltage step protocol. In all current-clamp recordings, recordings were made at resting membrane potential or without any current injection. Data analysis was performed using LabView. Myotube—hiCN coculture and live-cell imaging C2C12 myoblasts (ATCC) were expanded in DMEM supplemented with 20% FBS and then induced to form multinucleated myotubes by switching to medium containing 5% horse serum (Sigma). Purified hiCNs were then plated onto the myotube culture in C2 medium to induce the formation of neuromuscular junctions and myotube contractions. Live-cell imaging was performed using a Deltavision Deconvolution Microscope or an AMG EVOS Digital Inverted Microscope. Curare (tubocurarine hydrochloride, 50 μM, Sigma) was applied as indicated to block hiCN-induced rhythmic contraction. Neuromuscular junctions were visualized by confocal laser scanning microscopy after labelling with rhodamine-conjugated α-bungarotoxin (Invitrogen, 1:500) and immunostaining of SYT1 (DSHB, 1:200) and GFP (Invitrogen, 1:1,000). Statistical analysis All experiments were performed in triplicate at least twice unless otherwise indicated. Data are presented as mean±s.e.m. Statistical significance of differences between groups was determined using a two-tailed unpaired Student’s t -test. A P- value of <0.05 was considered significant. Accession codes : Microarray data have been deposited in Gene Expression Omnibus with accession code GSE45954 . How to cite this article: Liu, M.-L. et al. Small molecules enable neurogenin 2 to efficiently convert human fibroblasts into cholinergic neurons. Nat. Commun. 4:2183 doi: 10.1038/ncomms3183 (2013).